CSN- and CAND1-dependent remodelling of the budding yeast SCF complex Cullin–RING ligases (CRLs) are ubiquitin E3 enzymes with variable substrate-adaptor and -receptor subunits. All CRLs are activated by modification of the cullin subunit with the ubiquitin-like protein Nedd8 (neddylation). The protein CAND1 (Cullin-associated-Nedd8-dissociated-1) also promotes CRL activity, even though it only interacts with inactive ligase complexes. The molecular mechanism underlying this behaviour remains largely unclear. Here, we find that yeast SCF (Skp1–Cdc53–F-box) Cullin–RING complexes are remodelled in a CAND1-dependent manner, when cells are switched from growth in fermentable to non-fermentable carbon sources. Mechanistically, CAND1 promotes substrate adaptor release following SCF deneddylation by the COP9 signalosome (CSN). CSN- or CAND1-mutant cells fail to release substrate adaptors. This delays the formation of new complexes during SCF reactivation and results in substrate degradation defects. Our results shed light on how CAND1 regulates CRL activity and demonstrate that the cullin neddylation–deneddylation cycle is not only required to activate CRLs, but also to regulate substrate specificity through dynamic substrate adaptor exchange. Ubiquitin ligation to proteins requires a three-step enzymatic cascade involving E1, E2 and E3 enzymes. Activation of ubiquitin by the E1 leads to thioester bond formation between the active-site cysteine of the E1 and ubiquitin’s C-terminal glycine residue [1] , [2] . Ubiquitin is then transferred to the active-site cysteine of an E2 conjugating enzyme [3] , [4] , which binds to an E3 ligase. E3s recruit the substrate and catalyse isopeptide bond formation between ubiquitin and, most commonly, a lysine residue of the substrate [1] , [2] , [5] . Ubiquitylation often dramatically alters the properties of a protein and the best-characterized outcome is the degradation of poly-ubiquitylated substrates by the proteasome [3] , [4] , [5] . Cullin–RING complexes are modular E3 enzymes that consist of a cullin scaffold protein, which at its N terminus interacts with substrate-specificity modules, and at its C terminus binds to a small RING-finger protein (Rbx1 or Rbx2) that recruits the E2 enzyme [6] , [7] . Mammalian cells contain eight cullin proteins, Cul1, Cul2, Cul3, Cul4A, Cul4B, Cul5, Cul7 and Cul9/Parc [8] , while the S. cerevisiae genome encodes for three cullins, Cul1/Cdc53, Cul3 and Cul4/Rtt101. In yeast, Cul1/Cdc53 forms SCF (Skp1–Cdc53–F-box) Cullin–RING complexes together with the RING-finger protein Rbx1, the substrate adaptor Skp1 and one of 21 substrate receptor F-box proteins [6] . Different F-box proteins recruit different substrates to the ligase complex for ubiquitylation. SCF activity is tightly regulated. One level of regulation is modification of the cullin subunit with the ubiquitin-like protein Nedd8 (Rub1 in yeast, hereafter referred to as yNedd8) [9] , [10] . Nedd8 is the ubiquitin-like protein with the highest homology to ubiquitin and its major substrates are the cullins [11] , [12] . Neddylation activates Cullin–RING ligases (CRLs) by increasing the affinity of E2 to the ligase complex and by inducing structural flexibility, which allows the RING-finger protein to adopt a catalytically active conformation [13] , [14] . Deneddylation of Cullin–RING complexes is mediated by a deneddylase called the COP9 signalosome (CSN) [15] . The CSN is formed by eight proteins (CSN1-CSN8) and shows similarity to the lid of the 19S regulatory particle of the 26S proteasome [16] . The Nedd8 isopeptidase function is provided by CSN5, a JAMM metalloprotease, but all eight subunits are required for cullin deneddylation [17] . Even though deneddylation inactivates CRLs in vitro [18] , [19] , [20] , the CSN promotes ubiquitin ligase activity in vivo in various organisms [17] , [21] , [22] . This paradoxical behaviour can at least partially be explained by the fact that in cells constitutively neddylated complexes ubiquitylate their own subunits, leading to autodegradation [23] . Another CRL regulator, which also behaves like an inhibitor in vitro, but appears to be an activator in cells, is the protein CAND1 (Cullin-associated-Nedd8-dissociated-1). CAND1 interacts with Cullin–RING core complexes at both the N terminus, where it competes with the substrate adaptor for binding, and at the C terminus, where it masks the neddylation site [24] . Thus, CAND1 interaction with the cullin is mutually exclusive with substrate adaptor binding and neddylation [25] , [26] , [27] . On the basis of this observation, CAND1 has initially been suggested to sequester Cullin–RING core complexes and act as an inhibitor of ligase assembly and activation [24] . However, CAND1 loss-of-function mutations in Caenorhabditis elegans [28] and Arabidopsis thaliana [29] , [30] , [31] demonstrate that it is instead required for the activity of CRL ligases. To resolve this paradox, it has been proposed that instead of inactivating CRLs, CAND1 may ensure the formation of specific CRL complexes by allowing substrate adaptor exchange [32] , [33] . Changes in the abundance of some specific SCF complexes in CAND1-mutant A. thaliana and Schizosaccharomyces pombe indeed support this model [34] , [35] . We now directly show that CAND1 facilitates the remodelling of SCF ligases. We have identified a trigger, carbon-source switching, that allows rapid activation and inactivation of SCF E3s in yeast. We demonstrate that during inactivation, CAND1 releases substrate-adaptor and -receptor subunits from the SCF complex, but can only efficiently do so, when the complex is first deneddylated by the CSN. In CAND1- or CSN-mutant cells, substrate adaptors stay associated with the SCF, which results in a failure to form new complexes during reactivation and a delay in substrate degradation. CAND1 and the CSN thus cooperate to remodel SCF E3 ligases in yeast. Cdc53/Cul1 neddylation responds to changes in carbon source Budding yeast preferentially ferment glucose for ATP production, but the cells can adapt their metabolism to use non-fermentable carbon sources such as glycerol or ethanol. During glucose fermentation, yeast produce ethanol, which will be utilized as carbon source once glucose is depleted from the growth medium [36] ( Fig. 1a ). When cells again encounter glucose, they rapidly switch back to fermentation. 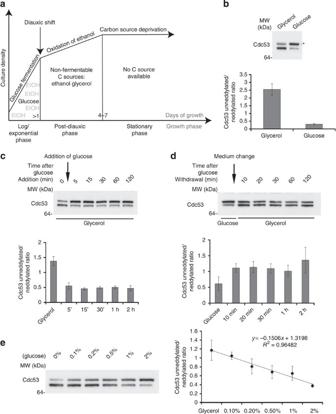Figure 1: The neddylation status of budding yeast Cdc53/Cul1 is sensitive to changes in carbon source. (a) Yeast carbon source utilization. Yeast ferment glucose during an exponential/log phase of growth and as a by-product, ethanol is released. Following glucose exhaustion, yeast switch from glucose fermentation to oxidative phosphorylation of non-fermentable carbon sources (for example, ethanol, glycerol). This metabolic switch is termed ‘diauxic shift’ and it marks an entry into a new phase of growth (post-diauxic phase). Complete exhaustion of carbon sources results in yeast entering stationary phase. (b) Yeast grown in glycerol-containing medium show markedly reduced neddylation of Cdc53/Cul1 as compared with cells grown on glucose. Asterisk indicates neddylated Cdc53/Cul1. Lower panel shows quantification as a mean of the ratio between unneddylated to neddylated Cdc53/Cul1. Error bars indicate s.d. (n=3). (c) Glucose was added to yeast grown in glycerol media, and the changes in neddylation were chased over time. Cdc53/Cul1 is fully neddylated already 5 min after glucose addition (quantification below as inFig. 1a; error bars indicate s.d. (n=3)). (d) Cells were grown in glucose-containing medium, pelleted, washed and resuspended in medium containing glycerol as sole carbon source. Neddylation of Cdc53/Cul1 was monitored over time. Change from glucose to glycerol medium induces a rapid reduction in Cdc53/Cul1 neddylation (quantification below as inFig. 1a; error bars indicate s.d. (n=3)). (e) Cells were grown in a medium containing the indicated concentration of glucose as sole carbon source. Cdc53/Cul1 neddylation increases linearly with the glucose concentration in the medium (quantification to the right; error bars indicate s.d. (n=3)). Figure 1: The neddylation status of budding yeast Cdc53/Cul1 is sensitive to changes in carbon source. ( a ) Yeast carbon source utilization. Yeast ferment glucose during an exponential/log phase of growth and as a by-product, ethanol is released. Following glucose exhaustion, yeast switch from glucose fermentation to oxidative phosphorylation of non-fermentable carbon sources (for example, ethanol, glycerol). This metabolic switch is termed ‘diauxic shift’ and it marks an entry into a new phase of growth (post-diauxic phase). Complete exhaustion of carbon sources results in yeast entering stationary phase. ( b ) Yeast grown in glycerol-containing medium show markedly reduced neddylation of Cdc53/Cul1 as compared with cells grown on glucose. Asterisk indicates neddylated Cdc53/Cul1. Lower panel shows quantification as a mean of the ratio between unneddylated to neddylated Cdc53/Cul1. Error bars indicate s.d. ( n =3). ( c ) Glucose was added to yeast grown in glycerol media, and the changes in neddylation were chased over time. Cdc53/Cul1 is fully neddylated already 5 min after glucose addition (quantification below as in Fig. 1a ; error bars indicate s.d. ( n =3)). ( d ) Cells were grown in glucose-containing medium, pelleted, washed and resuspended in medium containing glycerol as sole carbon source. Neddylation of Cdc53/Cul1 was monitored over time. Change from glucose to glycerol medium induces a rapid reduction in Cdc53/Cul1 neddylation (quantification below as in Fig. 1a ; error bars indicate s.d. ( n =3)). ( e ) Cells were grown in a medium containing the indicated concentration of glucose as sole carbon source. Cdc53/Cul1 neddylation increases linearly with the glucose concentration in the medium (quantification to the right; error bars indicate s.d. ( n =3)). Full size image During our studies of the yeast SCF complexes, we have noticed dramatic differences in the neddylation status of Cdc53/Cul1, when yeast are grown in either fermentable or non-fermentable carbon sources. In glucose (fermentable), the majority of Cdc53/Cul1 is neddylated, indicating that most molecules are engaged in active CRL complexes ( Fig. 1b ). However, the neddylation status of glycerol-grown yeast is greatly reduced, suggesting that the majority of Cdc53/Cul1 is inactive when non-fermentable carbon sources are metabolized ( Fig. 1b ). We have made identical observations in yeast supplied with ethanol ( Supplementary Fig. S1 ). Using LiCor quantification, we estimate that in glucose 76% of all cellular Cdc53/Cul1 is neddylated, whereas in glycerol this fraction drops to only 28% ( Fig. 1b ). Importantly, shifting cells from glycerol to glucose medium ( Fig. 1c ) or vice versa ( Fig. 1d ) rapidly induces this change in neddylation, indicating that it is mediated by a direct signalling event. Furthermore, the Cdc53/Cul1 neddylation status appears to increase linearly with the glucose concentration ( Fig. 1e ), suggesting that the fraction of Cdc53/Cul1 engaged in active complexes is highly sensitive to the available amount of glucose. Carbon-source switching specifically affects SCF complexes We next tested whether the change in neddylation is specific to Cdc53/Cul1, or whether it also affects other yeast cullins. Using yeast which express an endogenously GFP-tagged version of Cul3, we found that the Cul3 neddylation status was unaffected by carbon source ( Fig. 2a ). HA-Cul4/Rtt101 constitutively expressed from a centromeric plasmid even appeared slightly more neddylated during growth on glycerol ( Fig. 2a ), suggesting that the response to carbon source is specific to Cdc53/Cul1-based SCF complexes. 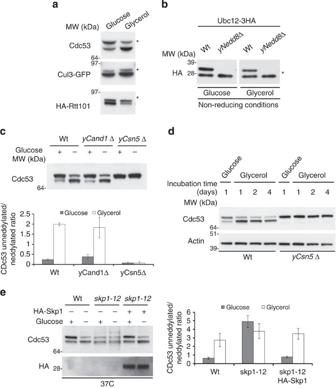Figure 2: Lack of fermentable carbon sources specifically impacts Cdc53/Cul1 neddylation in a CSN- and Skp1-dependent manner. (a) Western blots of Cdc53/Cul1, endogenously GFP-tagged Cul3 and HA-tagged Rtt101/Cul4 expressed from a centromeric plasmid in glucose or glycerol medium. Neddylation of each cullin is apparent as a more slowly migrating species (asterisks). Carbon source only affects neddylation of Cdc53/Cul1. (b) Charging of endogenously tagged Ubc12-3HA with yNedd8 (asterisk) is not affected by growth on glycerol. Experiment was performed under non-reducing conditions to preserve the thioester linkage between Nedd8 and the E2. (c) Cdc53/Cul1 neddylation in wild-type (WT),yCand1ΔandyCsn5Δcells in glucose (+) and glycerol-containing medium (−). Cells lacking yCand1 behave in a manner similar to WT with respect to their Cdc53/Cul1 neddylation, whereas cells devoid of Csn5 exhibit maximally neddylated Cdc53/Cul1 and do not respond to glucose withdrawal (quantification below). Error bars indicate s.d. (n=3). (d) Cdc53/Cul1 western blots from grown in glucose- or glycerol-containing medium for 1–4 days. In WT cells, reduction in Cdc53/Cul1 neddylation is sustained during prolonged growth on non-fermentable carbon source, while cells devoid of Csn5 maintain maximally neddylated cullin even after days of growth in glycerol. (e) Mutants of Skp1 no longer deneddylate Cdc53/Cul1 on non-fermentable carbon sources.Skp1-12temperature-sensitive mutants were shifted to the restrictive temperature (37 °C) in either glucose- or glycerol-containing media, and the neddylation of Cdc53/Cul1 was monitored by western blotting.Skp1-12mutants show decreased neddylation of Cdc53/Cul1 in glucose medium, and do not further reduce neddylation after switch to glycerol. This phenotype can be rescued by ectopically expressing WT Skp1 from a plasmid. Asterisk indicates neddylated form of Cdc53/Cul1. Quantification is depicted to the right. Error bars indicate s.d. (n=3). Figure 2: Lack of fermentable carbon sources specifically impacts Cdc53/Cul1 neddylation in a CSN- and Skp1-dependent manner. ( a ) Western blots of Cdc53/Cul1, endogenously GFP-tagged Cul3 and HA-tagged Rtt101/Cul4 expressed from a centromeric plasmid in glucose or glycerol medium. Neddylation of each cullin is apparent as a more slowly migrating species (asterisks). Carbon source only affects neddylation of Cdc53/Cul1. ( b ) Charging of endogenously tagged Ubc12-3HA with yNedd8 (asterisk) is not affected by growth on glycerol. Experiment was performed under non-reducing conditions to preserve the thioester linkage between Nedd8 and the E2. ( c ) Cdc53/Cul1 neddylation in wild-type (WT), yCand1Δ and yCsn5Δ cells in glucose (+) and glycerol-containing medium (−). Cells lacking yCand1 behave in a manner similar to WT with respect to their Cdc53/Cul1 neddylation, whereas cells devoid of Csn5 exhibit maximally neddylated Cdc53/Cul1 and do not respond to glucose withdrawal (quantification below). Error bars indicate s.d. ( n =3). ( d ) Cdc53/Cul1 western blots from grown in glucose- or glycerol-containing medium for 1–4 days. In WT cells, reduction in Cdc53/Cul1 neddylation is sustained during prolonged growth on non-fermentable carbon source, while cells devoid of Csn5 maintain maximally neddylated cullin even after days of growth in glycerol. ( e ) Mutants of Skp1 no longer deneddylate Cdc53/Cul1 on non-fermentable carbon sources. Skp1-12 temperature-sensitive mutants were shifted to the restrictive temperature (37 °C) in either glucose- or glycerol-containing media, and the neddylation of Cdc53/Cul1 was monitored by western blotting. Skp1-12 mutants show decreased neddylation of Cdc53/Cul1 in glucose medium, and do not further reduce neddylation after switch to glycerol. This phenotype can be rescued by ectopically expressing WT Skp1 from a plasmid. Asterisk indicates neddylated form of Cdc53/Cul1. Quantification is depicted to the right. Error bars indicate s.d. ( n =3). Full size image To exclude that the forward neddylation reaction is affected by growth on glycerol, we examined the charging of the yNedd8 E2 enzyme Ubc12 on fermentable and non-fermentable carbon sources. We detected no appreciable difference in both conditions ( Fig. 2b ), demonstrating that the neddylation pathway is functioning properly. Thus, the yeast metabolic status has a dramatic and specific effect on the activation of Cdc53/Cul1-based ligases, which allows us to use different carbon sources to rapidly manipulate SCF complexes. SCF deneddylation requires CSN and Skp1 but not yCand1 We next wanted to determine which SCF regulators are involved in mediating deneddylation upon carbon-source switching. The CSN is the only deneddylase in budding yeast, and we thus anticipated that the CSN also governs deneddylation during growth on glycerol. Indeed, cells lacking rri1 (yCsn5), the catalytic subunit of the CSN, no longer deneddylate Cdc53/Cul1 after carbon-source switching ( Fig. 2c ), even after days of growth in glycerol ( Fig. 2d ). As previous reports have suggested that the neddylation status of CRLs is directly regulated by the availability of substrates [37] , [38] , [39] , we next determined whether mutations of the substrate adaptor Skp1 or the substrate receptor F-box proteins would alter the response to non-fermentable carbon sources. When we examined a mutant of Skp1 ( skp1-12 ), we noticed that this strain displayed reduced Cdc53/Cul1 neddylation even in glucose, suggesting that functional Skp1 is required for wild-type levels of neddylation ( Fig. 2e ). Furthermore, the skp1-12 strain no longer responded to non-fermentable carbon sources with a reduction of neddylation, indicating Skp1 also has an important role in regulating changes in neddylation ( Fig. 2e ). We next examined deletion strains of all the non-essential F-box substrate receptor proteins, but none of them affected the neddylation response after carbon-source switching ( Supplementary Fig. S2 ). These results suggest that the availability of substrate may indeed signal changes in neddylation. However, as only mutations in Skp1 show a defect, which affects the association of all F-box proteins to the ligase complex, but not mutations of any single F-Box protein, the response is likely mediated by a combined effect of changes in the availability of many substrates. Because of its ability to only bind to non-neddylated cullin, we next hypothesized that CAND1 may also be involved in deneddylation of Cdc53/Cul1. However, deletion of the budding yeast CAND1 ortholog Lag2 (hereafter referred to as yCand1) [40] , [41] has no effect on Cdc53/Cul1 neddylation during carbon-source switching ( Fig. 2c ). Thus, yCand1 is not required for regulating deneddylation of SCF complexes, which is instead mediated by Skp1 and the CSN. Deneddylation does not alter interaction with yCand1 or CSN CAND1 has previously been suggested to sequester inactive CRL complexes. We thus reasoned that yCand1 might bind to the deneddylated form of Cdc53/Cul1, possibly keeping it inactive. However, when we immunoprecipitated Cdc53/Cul1 from glycerol and glucose-grown yeast, there was no apparent difference in the amount of coimmunoprecipitated yCand1 ( Fig. 3a ). This observation is consistent with what has been described for mammalian cullins after deneddylation through treatment with Nedd8 E1 inhibitor [42] , and it is thus unlikely that yCand1 is required to sequester non-neddylated complexes. 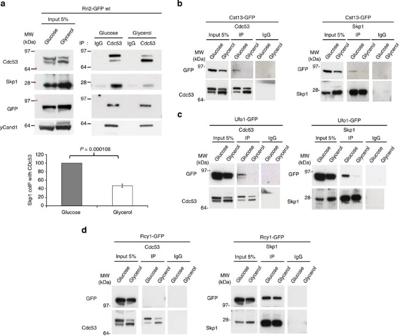Figure 3: Substrate adaptor/receptor modules dissociate from Cdc53/Cul1 and Skp1 during inactivation of the SCF. (a) Immunoprecipitation (IP) of Cdc53/Cul1 form cells grown in glucose or glycerol. There is no difference in the amount of coimmunoprecipitated yCand1 or Rri2-GFP (CSN subunit), while a significant loss of Skp1 substrate adaptor is detectable in glycerol. Quantification of the Skp1 signal below. Error bars indicate s.d. (n=4;P=0.000108 was calculated using Student’s two-tailedt-test). (b) Cdc53/Cul1 (left panel) and Skp1 (right panel) IP from glucose- or glycerol-grown yeast. Endogenously tagged Cst13-GFP association with Cdc53/Cul1 and Skp1 is significantly reduced in the presence of glycerol. (c) IP as inb, but from endogenously Ufo1-GFP-tagged strain. Growth on glycerol results in dissociation of Ufo1-GFP from Cdc53/Cul1 and Skp1, as assessed by its coimmunoprecipitation. (d) IP as inb, but from endogenously Rcy1-GFP-tagged strain. Rcy1 is an F-box protein that associates with Skp1 (right), but not Cdc53/Cul1 (left). For this non-SCF F-box protein interaction with Skp1, as assessed by its coimmunoprecipitation, is not affected by a change of carbon source. Figure 3: Substrate adaptor/receptor modules dissociate from Cdc53/Cul1 and Skp1 during inactivation of the SCF. ( a ) Immunoprecipitation (IP) of Cdc53/Cul1 form cells grown in glucose or glycerol. There is no difference in the amount of coimmunoprecipitated yCand1 or Rri2-GFP (CSN subunit), while a significant loss of Skp1 substrate adaptor is detectable in glycerol. Quantification of the Skp1 signal below. Error bars indicate s.d. ( n =4; P =0.000108 was calculated using Student’s two-tailed t -test). ( b ) Cdc53/Cul1 (left panel) and Skp1 (right panel) IP from glucose- or glycerol-grown yeast. Endogenously tagged Cst13-GFP association with Cdc53/Cul1 and Skp1 is significantly reduced in the presence of glycerol. ( c ) IP as in b , but from endogenously Ufo1-GFP-tagged strain. Growth on glycerol results in dissociation of Ufo1-GFP from Cdc53/Cul1 and Skp1, as assessed by its coimmunoprecipitation. ( d ) IP as in b , but from endogenously Rcy1-GFP-tagged strain. Rcy1 is an F-box protein that associates with Skp1 (right), but not Cdc53/Cul1 (left). For this non-SCF F-box protein interaction with Skp1, as assessed by its coimmunoprecipitation, is not affected by a change of carbon source. Full size image Furthermore, it has been reported that the non-neddylated inactive form of human Cul4 associates with the CSN [19] , [39] , and we thus tested whether this is also the case for the SCF in glycerol-grown yeast. However, the deneddylated cullin shows no increased association with the CSN, as determined by GFP immunoblotting of an endogenously GFP-tagged version of the CSN subunit Rri2 after Cdc53/Cul1 immunoprecipitation ( Fig. 3a ). Thus, although the SCF is deneddylated by the CSN, it does not stay associated with the complex. SKP1/F-box are released from the SCF during inactivation Although, we did not detect increased association of yCand1 and the CSN to non-neddylated Cdc53/Cul1 in glycerol-grown cells, there was a significant decrease in the amount of associated Skp1 substrate adaptor ( Fig. 3a ). Consistent with this observation, we also detected decreased interaction of two F-box proteins, Cst13 ( Fig. 3b , left panel) and Ufo1 ( Fig. 3c , left panel). This loss of F-box binding is not only seen with Cdc53/Cul1, but also directly with Skp1 after Skp1 immunoprecipitation ( Fig. 3b , right panels), suggesting that the loss of Skp1/F-box protein from CRLs goes hand in hand with dissociation of the Skp1-F-box heterodimer. The loss of Skp1-F-box interaction appears unique to F-boxes involved in CRLs, as it is not detected for Rcy1, a non-SCF F-box protein important for endocytic membrane trafficking ( Fig. 3d ) [43] . We concluded that CRL inactivation on non-fermentable carbon sources is associated with a loss of substrate adaptor and receptor binding. This reduction in Skp1/F-box binding could either be due to dissociation of substrate adaptor modules from existing ligase complexes, or due to the failure of newly synthesized Cdc53/Cul1 to associate with Skp1/F-box dimers. The latter possibility would require turnover of Cdc53/Cul1 during the experiment. We thus set out to determine the half-life of Cdc53/Cul1 in a timecourse experiment by treating cells with cycloheximide to stop protein translation. In glucose-grown cells, some degradation of Cdc53/Cul1 was apparent after 4 h of cycloheximide treatment ( Fig. 4a ). In glycerol-grown yeast, however, we detected no appreciable Cdc53/Cul1 degradation even 8 h after cycloheximide addition ( Fig. 4b ). As during our experiments cells are shifted to glycerol medium for 5–6 h before immunoprecipitation, we conclude that the reduction of Skp1/F-box binding represents a release of these proteins from inactivated complexes, rather than a failure of newly synthesized Cdc53/Cul1 to bind to Skp1/F-box heterodimers. 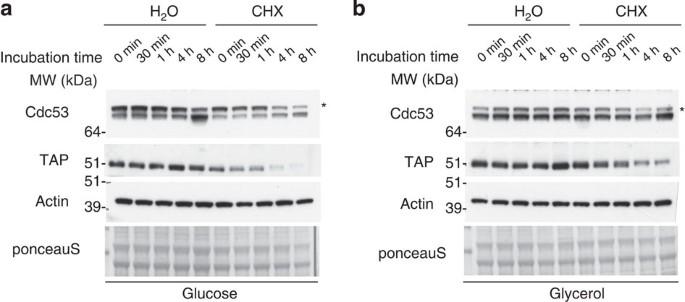Figure 4: Cycloheximide chase of Cdc53/Cul1 in glucose or glycerol medium. Cells were grown in glucose-containing medium (a) or glycerol-containing medium (b), and cycloheximide or vehicle control (water) was added to the medium to stop protein translation. Samples were taken at the indicated timepoints and the abundance of Cdc53/Cul1 was determined by western blotting. The unstable protein Ubc6-TAP (αTAP) was used as a positive control for successful cycloheximide treatment. In glucose, some degradation of Cdc53/Cul1 is apparent after 4 h of cycloheximide treatment, while Cdc53/Cul1 appears significantly more stable in glycerol medium and shows no apparent decrease in protein abundance even after 8 h of treatment. Asterisks indicate neddylated form of Cdc53. Figure 4: Cycloheximide chase of Cdc53/Cul1 in glucose or glycerol medium. Cells were grown in glucose-containing medium ( a ) or glycerol-containing medium ( b ), and cycloheximide or vehicle control (water) was added to the medium to stop protein translation. Samples were taken at the indicated timepoints and the abundance of Cdc53/Cul1 was determined by western blotting. The unstable protein Ubc6-TAP (αTAP) was used as a positive control for successful cycloheximide treatment. In glucose, some degradation of Cdc53/Cul1 is apparent after 4 h of cycloheximide treatment, while Cdc53/Cul1 appears significantly more stable in glycerol medium and shows no apparent decrease in protein abundance even after 8 h of treatment. Asterisks indicate neddylated form of Cdc53. Full size image Skp1 release from Cdc53/Cul1 requires yCand1 and CSN As substrate adaptor and CAND1 binding to CRLs is mutually exclusive, we reasoned that yCand1 might promote the Skp1-F-box release during SCF inactivation. Such a behaviour had previously been reported in a reconstituted in vitro system with immunoprecipitated mammalian proteins [37] . Using purified yeast proteins, we were able to dissociate Skp1–Cdc4 heterodimer from SCF Cdc4 with yCand1 ( Fig. 5a ), suggesting that a similar process could occur in cells. 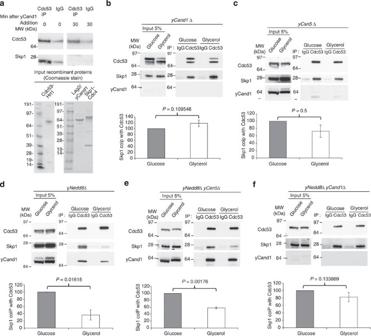Figure 5: The substrate adaptor Skp1 dissociates from Cdc53/Cul1 upon CRL inactivation in a yCand1- and CSN-dependent manner. (a)In vitrodissociation of Skp1–Cdc4 from Cdc53/Cul1. Cdc53–Skp1–Cdc4 were formed by mixing purified proteins (Coomassie gel below), and association of Skp1with Cdc53/Cul1 was determined by coimmunoprecipitation. Addition of yCand1 to preformed Cdc53–Skp1–Cdc4 complexes results in Skp1 release manifested by the loss of Skp1 coimmunoprecipitation with Cdc53/Cul1. (b) Cdc53/Cul1 immunoprecipitations (IPs) from yCand1-deleted cells. yCand1 deletion prevents glycerol-induced dissociation of Skp1 from Cdc53/Cul1. Quantification of the Skp1 signal is shown below. Error bars indicate s.d. (n=3;P=0.109546 was calculated using Student’s two-tailedt-test). (c) Cdc53/Cul1 IPs from yCsn5-deleted cells. yCsn5 deletion prevents Skp1 dissociation from Cdc53/Cul1 in glycerol medium. Quantification of the Skp1 signal below. Error bars indicate s.d. (n=4,P=0.5 was calculated using Student’s two-tailedt-test). (d) IPs of Cdc53/Cul1 from yNedd8-deleted cells. Lack of neddylation (yNedd8Δ) does not inhibit Skp1 dissociation from Cdc53/Cul1 in glycerol. Quantification of the Skp1 signal is shown below. Error bars indicate s.d. (n=3;P=0.01615 was calculated using Student’s two-tailedt-test). (e) IPs of Cdc53/Cul1 from yNedd8 and yCsn5 double-deleted cells. Simultaneous deletion of yNedd8 rescues the glycerol-induced Skp1 dissociation defect ofyCsn5Δcells. Quantification of the Skp1 signal is shown below. Error bars indicate s.d. (n=3;P=0.00176 was calculated using Student’s two-tailedt-test). (f) IPs of Cdc53/Cul1 from yNedd8 and yCand1 double-deleted cells. Simultaneous deletion of yNedd8 does not restore Skp1 dissociation from Cdc53/Cul1 inyCand1Δcells after a shift to glycerol. Quantification of the Skp1 signal is shown below. Error bars indicate s.d. (n=3;P=0.133869 was calculated using Student’s two-tailedt-test). Figure 5: The substrate adaptor Skp1 dissociates from Cdc53/Cul1 upon CRL inactivation in a yCand1- and CSN-dependent manner. ( a ) In vitro dissociation of Skp1–Cdc4 from Cdc53/Cul1. Cdc53–Skp1–Cdc4 were formed by mixing purified proteins (Coomassie gel below), and association of Skp1with Cdc53/Cul1 was determined by coimmunoprecipitation. Addition of yCand1 to preformed Cdc53–Skp1–Cdc4 complexes results in Skp1 release manifested by the loss of Skp1 coimmunoprecipitation with Cdc53/Cul1. ( b ) Cdc53/Cul1 immunoprecipitations (IPs) from yCand1-deleted cells. yCand1 deletion prevents glycerol-induced dissociation of Skp1 from Cdc53/Cul1. Quantification of the Skp1 signal is shown below. Error bars indicate s.d. ( n =3; P =0.109546 was calculated using Student’s two-tailed t -test). ( c ) Cdc53/Cul1 IPs from yCsn5-deleted cells. yCsn5 deletion prevents Skp1 dissociation from Cdc53/Cul1 in glycerol medium. Quantification of the Skp1 signal below. Error bars indicate s.d. ( n =4, P =0.5 was calculated using Student’s two-tailed t -test). ( d ) IPs of Cdc53/Cul1 from yNedd8-deleted cells. Lack of neddylation ( yNedd8Δ ) does not inhibit Skp1 dissociation from Cdc53/Cul1 in glycerol. Quantification of the Skp1 signal is shown below. Error bars indicate s.d. ( n =3; P =0.01615 was calculated using Student’s two-tailed t -test). ( e ) IPs of Cdc53/Cul1 from yNedd8 and yCsn5 double-deleted cells. Simultaneous deletion of yNedd8 rescues the glycerol-induced Skp1 dissociation defect of yCsn5Δ cells. Quantification of the Skp1 signal is shown below. Error bars indicate s.d. ( n =3; P =0.00176 was calculated using Student’s two-tailed t -test). ( f ) IPs of Cdc53/Cul1 from yNedd8 and yCand1 double-deleted cells. Simultaneous deletion of yNedd8 does not restore Skp1 dissociation from Cdc53/Cul1 in yCand1Δ cells after a shift to glycerol. Quantification of the Skp1 signal is shown below. Error bars indicate s.d. ( n =3; P =0.133869 was calculated using Student’s two-tailed t -test). Full size image Indeed, the release of Skp1 after a shift to non-fermentable carbon sources is inhibited in yCand1-deleted cells ( Fig. 5b ), demonstrating that substrate adaptor release from the CRL complex requires the activity of yCand1. As yCand1 only interacts with non-neddylated cullin, we further reasoned that deneddylation might be a prerequisite for Skp1 release. This is indeed the case, as cells carrying a deletion of Csn5, the catalytic subunit of the CSN, no longer efficiently dissociate Skp1 from the complex ( Fig. 5c ). However, this defect in Skp1 release, although still significant, is less pronounced than in yCand1Δ cells, suggesting that some yCand1-dependent release still occurs even if the cullin is fully neddylated. Importantly, no defect in Skp1 release is observed when neddylation is inhibited by deletion of yNedd8, demonstrating that only deneddylation, and not the cycle of neddylation and deneddylation, is required to liberate Skp1 from Cdc53/Cul1 ( Fig. 5d ). yNedd8 deletion rescues Skp1 release in yCsn5-mutant cells We speculated that the CSN is required to deneddylate Cdc53/Cul1 in order to allow efficient CAND1 binding and subsequent Skp1 release. If this was the case, then simultaneous deletion of yNedd8 should rescue the defect in yCsn5-deleted cells but not yCand1-deleted cells. This is indeed what we saw, as cells lacking both yNedd8 and CSN are able to release Skp1 from Cdc53/Cul1 ( Fig. 5e ), while yNedd8-/yCand1-doubly deleted cells were not rescued ( Fig. 5f ). These results demonstrate that yCand1 acts downstream of deneddylation in dissociating Skp1 from the cullin. We conclude that during inactivation of the SCF, the cullin first becomes deneddylated by the CSN, which allows yCand1 to release Skp1. Skp1 release is important for SCF function We next wanted to determine whether a failure to release Skp1 would have an effect on SCF function by testing whether degradation of Sic1 through the SCF Cdc4 is altered in yCand1Δ cells. Sic1 is a cyclin-dependent kinase inhibitor, which is degraded by the SCF at the G1/S transition of the cell cycle [44] . To determine differences in Sic1 degradation, we arrested cells with α-factor in G1 phase and monitored Sic1 levels after release into the cell cycle. However, we detected no difference between wild-type cells and cells lacking yCand1 in this assay, demonstrating that yCand1 is not important for the activity of this specific SCF ligase ( Fig. 6a ). 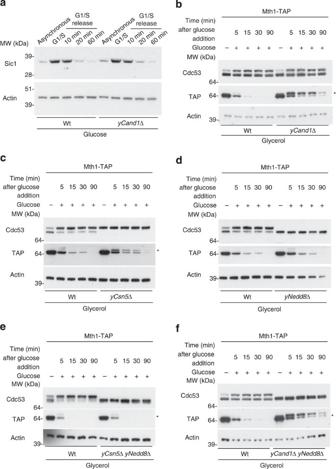Figure 6: Degradation of Mth1, but not Sic1, requires yCand1 and deneddylation by the CSN. (a) Degradation of Sic1 after α-factor arrest and release. Cells arrested at G1/S of the cell cycle were released into the cell cycle and the abundance of Sic1 was determined by western blotting. Sic1 is degraded with similar kinetics in wild-type (WT) cells and cells lacking yCand1. (b) Degradation of Mth1-TAP in WT cells and cells devoid of yCand1. Yeast strains were initially grown in glycerol. After glucose addition samples were taken at the indicated intervals and the abundance of an endogenously TAP-tagged form of Mth1 was determined by western blotting. In WT cells Mth1-TAP is rapidly degraded upon glucose addition and the glucose-induced phosphorylation of Mth1-TAP (asterisk) is hardly detectable. Deletion of yCand1 results in a strong accumulation of the phosphorylated form of Mth1-TAP, and a concomitant delay in Mth1-TAP degradation. (c) Mth1-TAP degradation is delayed inyCsn5Δcells, albeit less severely than in cells lacking yCand1. (d) Mth1-TAP degradation is not affected inyNedd8Δcells. (e) Simultaneous deletion of Nedd8 rescues the Mth1-TAP degradation defect in cells devoid of yCSN5. (f) Degradation of Mth1-TAP inyCand1Δcells is not rescued upon deletion of yNedd8 (yCand1Δ yNedd8Δ). Figure 6: Degradation of Mth1, but not Sic1, requires yCand1 and deneddylation by the CSN. ( a ) Degradation of Sic1 after α-factor arrest and release. Cells arrested at G1/S of the cell cycle were released into the cell cycle and the abundance of Sic1 was determined by western blotting. Sic1 is degraded with similar kinetics in wild-type (WT) cells and cells lacking yCand1. ( b ) Degradation of Mth1-TAP in WT cells and cells devoid of yCand1. Yeast strains were initially grown in glycerol. After glucose addition samples were taken at the indicated intervals and the abundance of an endogenously TAP-tagged form of Mth1 was determined by western blotting. In WT cells Mth1-TAP is rapidly degraded upon glucose addition and the glucose-induced phosphorylation of Mth1-TAP (asterisk) is hardly detectable. Deletion of yCand1 results in a strong accumulation of the phosphorylated form of Mth1-TAP, and a concomitant delay in Mth1-TAP degradation. ( c ) Mth1-TAP degradation is delayed in yCsn5Δ cells, albeit less severely than in cells lacking yCand1. ( d ) Mth1-TAP degradation is not affected in yNedd8Δ cells. ( e ) Simultaneous deletion of Nedd8 rescues the Mth1-TAP degradation defect in cells devoid of yCSN5. ( f ) Degradation of Mth1-TAP in yCand1Δ cells is not rescued upon deletion of yNedd8 ( yCand1Δ yNedd8Δ ). Full size image Next, we reasoned that instead of affecting SCF complexes at steady state, a failure to properly release Skp1 during SCF inactivation may only result in SCF defects during reactivation. We thus examined the activity of SCF Grr1 , an SCF complex, which is important to ubiquitylate the protein Mth1 when yeast cells encounter glucose. Upon glucose addition to the medium, the casein kinases Yck1 and Yck2 phosphorylate Mth1, which allows it to bind to the F-box substrate receptor Grr1 [45] . SCF Grr1 -dependent ubiquitylation of phosphorylated Mth1 then leads to rapid degradation by the proteasome ( Fig. 6b ) [45] . We found that in wild-type cells, the phosphorylated form of Mth1 remains virtually undetectable after glucose addition, due to its rapid ubiquitylation by SCF Grr1 ( Fig. 6b ). In yCand1-deleted cells, however, phospho-Mth1 is significantly stabilized, leading to a drastic delay in Mth1 degradation ( Fig. 6b ). We conclude that yCand1 is required for the degradation of Mth1 by regulating the activity of the SCF Grr1 complex during reactivation after glucose addition. We next reasoned that the Mth1 degradation defect is likely a direct consequence of the failure to release Skp1 during inactivation. If so, then Mth1 degradation should, just like Skp1 release, also require yCsn5 function, but not yNedd8. Mth1 degradation is indeed impaired in yCsn5Δ cells ( Fig. 6c ), and a clear stabilization of the phosphorylated form of Mth1 is detectable. Furthermore, consistent with the less pronounced defect in Skp1 release during SCF inactivation in yCsn5Δ cells, as compared with yCand1Δ cells, the delay in Mth1 degradation is also less pronounced. Finally, cells deleted for yNedd8 display normal Mth1 degradation ( Fig. 6d ), and simultaneous deletion of yNedd8 in yCsn5Δ cells restores Mth1 degradation, however, it does not do so in yCand1Δ cells ( Fig. 6e ). Thus, the genetic requirements for Mth1 degradation during SCF activation mirrors those of Skp1 release during inactivation, strongly suggesting that the Mth1 degradation defect is a consequence of the failure to release Skp1. Loss of yCand1 affects the association of Grr1 with the SCF We next examined the formation of the SCF Grr1 complex after glucose addition to determine how a defect in Skp1 release may affect Mth1 degradation. As Mth1 is degraded rapidly after exposure to the signal ‘glucose’, we hypothesized that this quick response might require fast association of newly formed Skp1–Grr1 substrate-specificity modules, with already existing Cullin–RING core complexes. In the absence of yCand1, the binding site on the cullin may still be occupied with old substrate adaptor modules, which could prevent the formation of new complexes. To test this hypothesis, we examined binding of the F-box protein Grr1 to Skp1 and to Cdc53/Cul1 after addition of the glucose to cells. In Skp1 immunoprecipitates from both wild-type and yCand1Δ cells, an increased association of Grr1 to Skp1 was apparent already after 5 min of glucose addition to the medium ( Fig. 7a ). In wild-type cells, this binding to Skp1 translated into a rapid induction of Grr1 association with Cdc53/Cul1, demonstrating that SCF Grr1 complexes are formed upon glucose addition ( Fig. 7c , left panel). In yCand1Δ cells, however, Grr1 was already associated with Cdc53/Cul1 even in the absence of glucose ( Fig. 7c ). This basal association is likely a reflection of the failure to release Skp1/F-box modules during inactivation of the complex. Importantly, there was no increase in Grr1 associated with Cdc53/Cul1 after glucose addition, even though the amount of Grr1 bound to Skp1 increased. This indicates that although Skp1–Grr1 complexes are formed, they are formed independent of Cdc53/Cul1 and are not efficiently incorporated into SCF ligases, presumable because ‘old’ substrate-specificity modules occupy Cdc53/Cul1. The non-cullin-bound Skp1–Grr1 substrate adaptor complexes likely still interact with the substrate, which would shield Mth1 from ubiquitylation by the E3. We eventually detected a slight increase in Grr1 association with Cdc53/Cul1 after 30 min of glucose exposure ( Fig. 7c ), suggesting that the binding is delayed but not entirely inhibited. 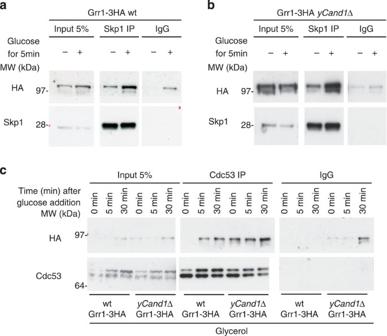Figure 7: yCand1 is required for the association of Skp1–Grr1 to the cullin–RING core after glucose addition. Skp1 immunoprecipitations (IPs) from wild-type (WT;a) or yCand1-deleted cells (b) carrying endogenously tagged Grr1-3HA. In glycerol, low amounts of Grr1-3HA are associated with Skp1 in both strains. Within 5 min of glucose stimulation, an increase in Grr1-3HA bound to Skp1 is apparent in both WT andyCand1Δcells. (c) Cdc53/Cul1 IPs from WT or yCand1-deleted cells carrying endogenously tagged Grr1-3HA. In WT cells, Grr1-3HA does not coimmunoprecipitate with Cdc53/Cul1 in glycerol medium. Five minutes upon glucose stimulation an interaction betweenGrr1-3HA and Cdc53/Cul1 is detectable, and this interaction is also maintained 30 min after glucose addition. In cells devoid of yCand1, Grr1-3HA association with Cdc53/Cul1 is detectable even in glycerol media, but there is no increase in association 5 min after glucose addition. A slight increase is detectable 30 min after glucose was supplied to the cells. Figure 7: yCand1 is required for the association of Skp1–Grr1 to the cullin–RING core after glucose addition. Skp1 immunoprecipitations (IPs) from wild-type (WT; a ) or yCand1-deleted cells ( b ) carrying endogenously tagged Grr1-3HA. In glycerol, low amounts of Grr1-3HA are associated with Skp1 in both strains. Within 5 min of glucose stimulation, an increase in Grr1-3HA bound to Skp1 is apparent in both WT and yCand1Δ cells. ( c ) Cdc53/Cul1 IPs from WT or yCand1-deleted cells carrying endogenously tagged Grr1-3HA. In WT cells, Grr1-3HA does not coimmunoprecipitate with Cdc53/Cul1 in glycerol medium. Five minutes upon glucose stimulation an interaction betweenGrr1-3HA and Cdc53/Cul1 is detectable, and this interaction is also maintained 30 min after glucose addition. In cells devoid of yCand1, Grr1-3HA association with Cdc53/Cul1 is detectable even in glycerol media, but there is no increase in association 5 min after glucose addition. A slight increase is detectable 30 min after glucose was supplied to the cells. Full size image It consequently appears that although the Skp1–Grr1 heterodimer is readily formed upon addition of glucose, it cannot be incorporated into the Cdc53/Cul1 complex in the absence of yCand1. We propose that this incorporation defect is likely a direct consequence of the failure to release substrate-adaptor/-receptor complexes during inactivation. Thus, the CSN and CAND1 cooperatively promote substrate-adaptor/-receptor exchange, giving SCF complexes the ability to rapidly respond to signals that require fast ubiquitylation of new substrates. In recent years, CAND1 has been suggested on numerous occasions to act as an exchange factor for substrate adaptors of CRLs [33] , [38] , [46] . Using the yeast SCF ligases, we have now been able to show that this is indeed the case. Our analysis was greatly aided by the fact that carbon-source switching induces bulk activation and inactivation of the Cdc53/Cul1-based ligases in yeast. To our knowledge, this is the first instance of a CRL complex to respond so dramatically to an extracellular stimulus. There have been other reports of changes in cullin neddylation upon different signals, but they appear less pronounced than what we see with Cdc53/Cul1 in yeast. For example, mammalian Cul4 is released from the CSN upon UV-induced DNA damage [19] , and the SCF in plants becomes more neddylated after exposure to light [47] . It would be interesting to see whether in these instances CAND1 is also involved in regulating ligase assembly. Although CAND1 and the CSN promote substrate adaptor release during SCF inactivation in yeast, the initial signal that triggers inactivation remains unclear. In the future it will be important to understand the molecular mechanism behind the SCF sensitivity to carbon-source switching. As the inactivation is closely coupled to deneddylation of the SCF complex by the CSN, it is conceivable that the association of the SCF with the CSN is regulated directly by post-translational modifications. However, an increasing body of evidence suggests that neddylation of CRL complexes is governed by substrate binding to the CRL [37] , [38] , [39] . Similarly, our data also support an involvement of substrate in regulating the Cdc53/Cul1 neddylation response to carbon-source switching. We show that skp1-12 mutants display neddylation defects and are no longer able to dynamically change the Cdc53/Cul1 neddylation state. If the availability of substrate is indeed driving the changes in neddylation, then it is conceivable that during growth on glucose many more substrates require ubiquitylation by the SCF than during growth on glycerol. The amount of active neddylated complexes would then be proportional to the amount of available substrates, as the substrate would directly trigger the activation of its own E3 complex. If this is indeed the case, then SCF ligases that can no longer bind to substrate should stay deneddylated and inactive. However, our data show that even though Skp1–Grr1 is no longer efficiently recruited to the complex in yCand1-mutant cells, the SCF still becomes neddylated when glucose is added to the medium. Although this neddylation could be triggered by other SCF substrates that are insensitive to CSN-/CAND1-dependent regulation, it is also possible that substrate-independent factors have an important role in SCF regulation in yeast. Our data in yeast demonstrate that CAND1 is an exchange factor for CRL substrate adaptor modules. However, it appears that under most conditions this activity is not essential for ligase function. For example, we show that the SCF Cdc4 complex is not affected by a lack of yCand1. Also, in C. elegans CAND1 mutations only show subtle phenotypes that are likely due to the loss of function of one specific CRL complex, the SCF Lin23 (ref. 28 ). Furthermore, short interfering RNA to CAND1 in mammalian cells has very little effect on the abundance of a range of CRL substrates [42] . CAND1 may thus only regulate the formation of specific complexes, or there could be redundant systems that ensure CRL formation. For example, CAND1 may only become important when there are not enough inactive Cullin–RING core ligases present to form new complexes. There is evidence that inactive CRLs awaiting activation exist in the cell. Cul4 in mammalian cells, for example, is mostly inactive and bound to the CSN. Active Cul4 complexes are only formed upon binding of a substrate [39] . One could imagine a similar situation for other cullins, where a significant pool exists in an inactive form. An exchange factor for substrate adaptors would then in most cases not be necessary, as any new substrate receptor modules could first activate dormant CRL core complexes. Also, even when most of the CRL core complexes are engaged with substrate adaptor subunits, a CAND1-promoted formation of new complexes may not be necessary in all instances. Instead, it could be sufficient for most ligases to be formed with newly synthesized cullins instead of exchanging the substrate adaptors of already existing CRLs. Thus, CAND1 may only be critical in situations where there are little cullin reserves and the cell has to rapidly respond to a signal with the formation of a new complex. In the case of Mth1, this is indeed the case, as here during growth in glucose medium, most of Cdc53/Cul1 is active and bound to Skp1–F-box proteins. Although deneddylation ensues during the shift to glycerol, the lack of yCand1 prevents the dissociation of substrate adaptor subunits. This keeps most of the Cdc53/Cul1 core complexes sequestered from newly formed Skp1–Grr1 heterodimers, when the cell has to rapidly respond to glucose addition with degradation of Mth1. Our observations also raise an important question about the role of the neddylation–deneddylation cycle for CRL ligase activity. The neddylated form of a CRL complex is thought to be the active version, which is confirmed by in vitro experiments, where neddylated complexes are significantly better E3 ubiquitin ligases [19] . In cells, however, deneddylation is also important for E3 activity [32] . This observation, commonly referred to as the CSN paradox, is explained by the fact that hyperactive CRLs ubiquitylate their own subunits, effectively inactivating themselves by autodegradation [20] , [48] . Our data now suggest that defects in deneddylation also prevent the formation of new CRL complexes due to a lack of CAND1-mediated substrate adaptor exchange, which likely accounts for some of the CRL defects observed in CSN-defective cells. Our observations also add another level of complexity to the regulation of CRLs by neddylation. On the basis of our data, Nedd8 not only activates complexes by enhancing their E3 ligase activity, but also has a pivotal role in governing the association and exchange of substrate adaptors by regulated deneddylation. It has always been puzzling why CRLs need an additional level of regulation of ligase activity via a ubiquitin-like molecule, whereas other E3 ubiquitin ligases can do without. It is thus tempting to speculate that the original function of the Nedd8 cycle is not in activating CRL ligases, but in regulating the association and dissociation of substrate adaptors. Yeast growth conditions Yeast strains used are listed in Supplementary Table S1 . Standard yeast growth conditions and genetic manipulations were used in this study [26] . For glucose starvation of yeast, cultures were pelleted, washed three times in a large volume of prewarmed YPA+3% glycerol (YPAGly) media and resuspended in a final volume of YPAGly for indicated timepoints. For supplementation of glucose-starved yeast with glucose, cells were first inoculated into YPAD media and incubated overnight at 30 °C until a OD 600 of ~7–8 was obtained. Yeast were then diluted with YPAGly until a OD 600 of 0.4 was obtained, and incubated for 5 h at 30 °C before the addition of 2% glucose directly in to the culture for indicated timepoints. Antibodies The following antibodies were used: anti-Cdc53 (yN300, Santa Cruz Biotechnology), anti-TAP (Sigma Aldrich), anti-actin (C4, Millipore), anti-GFP (Roche), anti-HA (6E2, Cell Signalling Technology), anti-Sic1 (kindly provided by Prof. Mike Tyers), anti-yCand1 was kindly provided by Prof. Matthias Peter, anti-Skp1 (raised in sheep against residues 95-C-terminal end) and anti-Cdc53 (raised in sheep against residues 1–228). G1/S cell cycle arrest To arrest yeast in G1/S phase of the cell cycle, exponentially growing yeast were first washed twice in sterile H 2 O to remove Bar1, which degrades α-factor. Pellets were resuspended in an appropriate medium and treated with 5 μg ml −1 α-factor (Sigma Aldrich) or vehicle control until cells started to show ‘shmoo’ morphology, and <95% were budded. To release cells from G1/S, yeast were washed three times in prewarmed medium and resuspended in a final volume of the same medium for indicated timepoints. G1/S arrest was monitored through immunodetection of endogenous Sic1. Yeast protein extract preparation Cells were precultured at 30 °C in YPAD until OD 600 of ~7–8. Cultures were either diluted into 500 ml YPAD to OD 600 =0.05 or into 500 ml YPAGly to OD 600 =0.4, and incubated at 30 °C for ~8 h. Three millilitre of the culture was taken for the preparation of the trichloroacetic acid or tricarboxylic acid protein sample as an input. The remaining culture was harvested through centrifugation at 4,200 r.p.m. for 55 min at 4 °C. Pellets were washed in ice-cold water and centrifuged at 3,100 r.p.m. for 5 min at 4 °C. Pellets were resuspended in ice-cold lysis buffer (10 mM Hepes (pH 7.9), 10 mM KCl, 1.5 mM MgCl 2 , 5 mM iodoacetamide, PhosStop phosphatase inhibitor (Roche), complete EDTA-free protease inhibitor (Roche)), flash frozen in liquid nitrogen and lysed mechanically using Freezer Mill 6770 Spex Sample Prep. Protein lysates were cleared from cell debris through ultracentrifugation at 50,000 r.p.m. for 20 min at 4 °C and then at 13,300 r.p.m. for 20 min at 4 °C. Protein concentration of the lysate was established using BCA Protein Assay Kit (Pierce). Immunoprecipitation from protein extracts Four miligram of protein was mixed with 40 μl of Protein G Agarose slurry (Pierce) equilibrated in lysis buffer. For Cdc53 immunoprecipitations, 20 μg of Cdc53 antibody raised against residues 1–228 was used, whereas for Skp1 immunoprecipitation, 20 μg of Skp1 antibody raised against residue 95-C terminus was used. Twenty microgram of preimmune sheep IgG was used to control for unspecific protein binding. Samples were incubated overnight at 4 °C, subsequently centrifuged at 3,000 r.p.m. for 4 min and washed four times in ice-cold wash buffer (10 mM Hepes (pH 7.9), 300 mM KCl, 2 mM CHAPS, 5 mM iodoacetamide, PhosStop phosphatase inhibitor (Roche), complete EDTA-free protease inhibitor (Roche)). Proteins were eluted off the beads by boiling samples for 10 min in 3 × reducing SDS sample buffer. Purification of recombinant proteins yCand1 was expressed in E. coli as a GST-fusion protein, purified over GSH-Sepharose and recovered by cleaving off the tag with Prescission Protease. It was then dialysed into 50 mM HEPES (pH 7.5), 10% glycerol, 150 mM NaCl and 1 mM DTT. The cloning and purification of Cdc53/Hrt1 was described by Lee et al [27] . The identity of all proteins was confirmed by mass spectrometry. Skp1–Cdc4 heterodimer was a kind gift from Prof. Mike Tyers. Immunoprecipitation of purified SCF complexes Three point two picomoles of purified Cdc53/Hrt1 and 3.2 pmoles of Skp1–Cdc4 were mixed in the reaction buffer (10 mM Hepes (pH 7.9), 10 mM KCl, 1.5 mM MgCl 2 ) for 30 min at room temperature to allow complex formation. Following addition of 32 pmoles of recombinant yCand1, samples were incubated for another 30 min. For Cdc53 immunoprecipitations, 2 μg of Cdc53 antibody (raised against residues 1–228) or preimmune sheep IgG was added with 10 μl of Protein G Agarose slurry (Pierce). After 30-min incubation at room temperature, samples were washed four times in wash buffer (10 mM Hepes (pH 7.9), 300 mM KCl, 2 mM CHAPS), eluted off the beads by boiling in 3 × reducing SDS sample buffer and analysed by western blotting. Quantitative analysis of immunoblots Quantitative analysis of immunoblots was performed using Odyssey Infrared Imaging System (Li-COR). Immunodetection of Cdc53 was analysed using IRDye 800CW goat anti-rabbit secondary antibody (Li-COR). Intensity of Cdc53-reactive bands was quantified based on fluorescent output of secondary antibodies with Li-COR Odyssey software. Statistical analysis Data are presented as means±s.d. Where indicated, two groups were compared using Student’s two-tailed t -test. How to cite this article: Zemla, A. et al . CSN- and CAND1-dependent remodelling of the budding yeast SCF complex. Nat. Commun. 4:1641 doi: 10.1038/ncomms2628 (2013).